HIF-1 stabilization in T cells hampers the control ofMycobacterium tuberculosisinfection The hypoxia-inducible factors (HIFs) regulate the main transcriptional pathway of response to hypoxia in T cells and are negatively regulated by von Hippel-Lindau factor (VHL). But the role of HIFs in the regulation of CD4 T cell responses during infection with M. tuberculosis isn’t well understood. Here we show that mice lacking VHL in T cells ( Vhl cKO ) are highly susceptible to infection with M. tuberculosis , which is associated with a low accumulation of mycobacteria-specific T cells in the lungs that display reduced proliferation, altered differentiation and enhanced expression of inhibitory receptors. In contrast, HIF-1 deficiency in T cells is redundant for M. tuberculosis control. Vhl cKO mice also show reduced responses to vaccination. Further, VHL promotes proper MYC-activation, cell-growth responses, DNA synthesis, proliferation and survival of CD4 T cells after TCR activation. The VHL-deficient T cell responses are rescued by the loss of HIF-1α, indicating that the increased susceptibility to M. tuberculosis infection and the impaired responses of Vhl -deficient T cells are HIF-1-dependent. Tuberculosis (TB), caused by infection with Mycobacterium tuberculosis , remains a leading public health problem. While most individuals infected with M. tuberculosis remain asymptomatic, in 2018 10 million individuals fell ill with this disease and 1.5 million died [1] . Why M. tuberculosis occurs only in some individuals is only partially understood. The risk of developing TB increases during HIV and M. tuberculosis co-infection suggesting that impairment of CD4 T cell-mediated immune responses reactivates the asymptomatic infection [2] . The central role for CD4 T cells in protective immunity against TB is also evidenced by the extreme susceptibility of animals lacking CD4 T cells [3] . T H 1 immune responses that involve cellular effector mechanisms such as IFN-γ mediated macrophage activation are utilized by the host to counteract mycobacterial infections [4] , [5] , [6] , [7] . Bacille Calmette–Guérin (BCG) the only TB vaccine shows a variable efficiency against pulmonary TB in adults [8] , and a better vaccine against M. tuberculosis is urgently needed. Correlates of protective immune responses to M. tuberculosis infection in humans remain undefined. Understanding the detailed molecular regulation of T cell functions in the lung is paramount for building a strategy for vaccine induced protection against TB. Survival, activation, and effector function of T cells is fundamentally linked to cellular metabolic programming [9] . A number of transcription factors have been implicated in the regulation of T cell metabolism and the T cell responses following activation [10] . Hypoxia is a hallmark trait of inflamed tissues. The hypoxic stress response is largely governed by hypoxia-inducible factors HIF-1α and HIF-2α, that heterodimerize with HIF-1β and serve as the central sensor of oxygen tension in all cells. HIFs are highly relevant to the proper function of different immune cell populations including T cells [11] . In normal oxygen tensions, the HIF-α proteins are hydroxylated by prolyl hydroxylase domain proteins (PHD or EGLN proteins). These modifications are recognized by the von Hippel Lindau tumor suppressor protein (VHL), an E3 ubiquitin ligase that drives the degradation of the HIF-α subunits [12] , [13] , [14] . HIF-1 and HIF-2 drive a metabolic reprogramming through the upregulation of glycolytic metabolism and the suppression of oxygen consumption by mitochondria [15] . In T cells, signals mediated by T cell antigen receptors (TCRs), cytokines and innate immune receptors have been shown to activate HIF-pathways even under normal oxygen tension [11] . Constitutive HIF activity achieved by conditional deletion of Vhl or Phd (s) had been shown to modulate the effector functions, the differentiation, and the expression of inhibitory receptor in CD4 and CD8 T cells, improving the control of tumors and viral infections [16] , [17] , [18] . Here, we studied the role of HIFs in the regulation of T cells during M. tuberculosis infection. In contrast to previous observation that VHL deficiency enhances effector responses of T cells, mice with VHL-loss in T cells ( Vhl cKO ) showed a dramatically increased susceptibility to infection with M. tuberculosis by failing to accumulate M. tuberculosis -specific CD4 and CD8 T cells in the lungs. Mutant T cells showed reduced levels of differentiation markers, increased expression of inhibitory receptors and low IFN-γ secretion. In contrast HIF-1-deficiency in T cells was redundant for protection against M. tuberculosis infection. We showed that VHL promoted CD4 T cell activation after T-cell receptor (TCR) stimulation. We demonstrated that the impaired TCR-mediated responses, the increased susceptibility to M. tuberculosis and the defect in mounting responses to immunization of Vhl cKO CD4 T cells are due to HIF-1 stabilization. VHL, but not HIF-1 expression in T cells is critical for the control of M. tuberculosis infection in mice We studied the role of VHL and HIF-1 in T cells in the outcome of infection with 250 M. tuberculosis using Vhl fl/fl cd4 cre ( Vhl cKO ) and Hif1a fl/fl dlck cre ( Hif1a cKO ) mice. Lungs and spleens from Vhl cKO mice at 4, 6 and 8 weeks after aerosol infection all showed increased levels of M. tuberculosis as compared to those from Vhl fl/fl controls (WT) (Fig. 1a, b ). Vhl cKO mice lost weight as compared to WT controls (Fig. 1c ). The lungs from M. tuberculosis -infected Vhl cKO mice showed lesions engaging a larger area of the lung as compared to those from controls (Fig. 1d ). Vhl cKO mice also showed decreased cumulative survival after M. tuberculosis infection (Fig. 1e ). The titers of M. tuberculosis in lungs and spleens from Hif1a cKO and Hif1a fl/fl littermates (WT) were similar (Fig. 1f ). The lesion severity in lungs from Hif1a cKO and WT mice was similar (Supplementary Fig. 1a ), and no mortality was observed in these groups. Fig. 1: VHL expression in T cells is critical for the control of M. tuberculosis infection in mice. a , b Vhl cKO and WT mice were infected via aerosol with 250 M. tuberculosis and sacrificed at indicated time points after infection. The log 10 CFU in the lung ( a ) and spleen ( b ) of individual mice ( n WT = 10, 9, 12; n Vhl cKO = 9, 9, 10 mice at 4, 6 and 8 weeks post infection (w.p.i.) respectively) are represented. c The weight change with respect to the uninfected group mean (day 0) during infection with M. tuberculosis of Vhl cKO and WT mice ( n = 11 per group) is depicted. d Representative micrographs from hematoxylin-eosin-stained paraffin lung sections from Vhl cKO and WT mice 8 w.p.i. with M. tuberculosis (bar: 400 μm). e The cumulative mortality of Vhl cKO and WT mice ( n = 9 per group) after M. tuberculosis infection is depicted. f The log 10 CFU in the lungs and spleens of Hif1a cKO ( n = 11) and WT ( n = 9) mice 8 w.p.i. with M. tuberculosis are shown. g – i The representative dot plots of CD4 and CD8 (gated on T cells) in the lungs of Vhl cKO and WT mice before and 8 w.p.i. with M. tuberculosis ( g ), and the frequency of CD4 ( h ) and CD8 ( i ) T cells in the lungs (WT n = 4, 4, 6, 8 and Vhl cKO n = 4, 5, 6 and 8 mice at 0, 4, 6 and 8 w.p.i. respectively). j , k The frequency of CD4 and CD8 T cells in the lungs of Hif1a cKO and WT mice before ( n = 4 per group) and 8 w.p.i. ( n = 5 per group) are depicted. l , m The frequency of CD4 in spleens ( l ) and mediastinal lymph nodes ( m ) before and 8 w.p.i. with M. tuberculosis are shown ( Vhl cKO n = 4, 7 and WT n = 4, 4 mice at 0 and 8 w.p.i., respectively). Rag2 −/− mice were administered i.v. with either 2.10 6 Vhl cKO or WT CD4 T cells ( n = 6) or left untreated 3 days after M. tuberculosis infection. The log 10 CFU in the lungs and spleens ( n ) ( n = 8 animals per group) and number of CD4 T cells ( o ) in lungs ( n = 6 mice per group) 4 w.p.i. Each symbol represents one mouse, and the data are presented as the mean ± s.e.m. The p -values were calculated using either a two-tailed unpaired t test with Welch’s correction for no homoscedasticity and FDR approach for multiple comparison ( a , b , f , h – m , o ), a one-way ANOVA with Welch’s correction ( n ), a 2-way ANOVA with Sidak’s multiple comparison test ( c ), or a χ 2 test ( e ). Source data are provided as a Source Data file. Full size image Next, we evaluated the impact of the HIF-1 and VHL-deficiency on the numbers, frequencies and phenotype of pulmonary T cells during M. tuberculosis infection. We found that the frequencies and numbers of T cells in lungs from Hif1a cKO , Vhl cKO and WT mice before and after M. tuberculosis infection were similar (Supplementary Fig. 1b–d ). However, lungs from M. tuberculosis -infected Vhl cKO mice showed a reduced frequency of CD4 T cells at 4, 6 and 8 weeks after infection when compared to WT mice (Fig. 1g, h ). The frequency of lung CD8 T cells at 8, but not at 4 and 6 weeks after infection, was decreased in Vhl cKO mice (Fig. 1g, i ). Instead, the frequency and numbers of Vhl cKO CD4-CD8- (DN) T cells, consisting of a majority of γδT cells was higher in Vhl cKO than in WT controls (Supplementary Fig. 1e–h ). The frequencies of CD4, CD8 and DN T cells in lungs from Hif1a cKO and WT mice before or after infection with M. tuberculosis were instead similar (Fig. 1j, k and Supplementary Fig. 1i ). Vhl cKO mice showed low levels of CD4 T cells in spleens and mediastinal lymph nodes (MLN) at 8 weeks after infection (Fig. 1l, m ). Of importance, the frequencies of CD4 and CD8 T cells in lungs, spleens and MLN from uninfected Vhl cKO and WT mice was similar (Fig. 1h, i, l, m ). The total cell numbers in the MLNs in WT and Vhl cKO mice were similar, whereas MLN CD4 T cells numbers were reduced in Vhl cKO M. tuberculosis infected mice when compared to controls (Supplementary Fig. 1j, k ). CD4 T cells are critical for the control of M. tuberculosis infection [3] , [19] . To address whether VHL-deficiency in CD4 T cells hampers their protective capacity against M. tuberculosis , naïve Vhl cKO or WT CD4 T cells were transferred to Rag2 − /− mice 3 days after infection with M. tuberculosis . The bacterial load in lungs and spleens from mice 4 weeks after transfer with WT CD4T cells was lower than in those from non-transferred infected controls (Fig. 1n ). Rag2 −/− mice transferred with Vhl cKO CD4 T cells showed increased bacterial loads in lungs and spleens and lower number of CD4 T cells in the lung when comparing to mice transferred with WT CD4 T cells (Fig. 1n, o and Supplementary Fig. 1l , m). Thus, transfer of Vhl cKO CD4 T cells do not confer protection against M. tuberculosis infection. Low levels of mycobacteria-specific T cells in lungs of Vhl cKO infected mice The levels of M. tuberculosis -specific CD4 and CD8 T cells in the lungs from Vhl cKO , Hif1a cKO and WT mice were then compared. The frequency of ESAT6 1-20 -tetramer binding CD4 T cells in the lungs of Vhl cKO after infection with M. tuberculosis was reduced when compared to that of WT mice (Fig. 2a, b ). Instead, the frequencies of ESAT6-tetramer binding cells in lungs from M. tuberculosis - infected Hif1a cKO and WT mice were similar (Fig. 2c ). Fig. 2: Reduced accumulation of mycobacteria-specific T cells in the lungs of M. tuberculosis infected Vhl cKO mice. a Representative dot plots of tetramer ESAT-6-binding CD4 T cells in the lungs from Vhl cKO and WT mice 8 weeks post infection (w.p.i.) with M. tuberculosis are depicted. b The percentage of tetramer ESAT-6-binding CD4 T cells in the lungs of Vhl cKO and WT mice (WT n = 5, 5, 7 and Vhl cKO n = 5, 7, 7 mice at 4, 6 and 8 w.p.i.) are displayed. c Percentage of tetramer ESAT-6 + CD4 T cells in the lungs of Hif1a cKO ( n = 5) and WT ( n = 5) mice 8 w.p.i. ( d , e ) Dot plots ( d ) and the frequency of tetramer TB10.4-binding CD8 T cells ( e ) in the lungs from Vhl cKO ( n = 5, 6) and WT mice ( n = 5, 7 animals at 4 and 8 w.p.i., respectively) are depicted. f The frequency of tetramer TB10.4-binding lung Hif1a cKO ( n = 5) and WT ( n = 5 mice) CD8 T cells at 8 w.p.i. is depicted. g , h The frequencies of IFN-γ secreting CD4 ( g ) and CD8 ( h ) T cells from Vhl cKO ( n = 9) and WT ( n = 9) mice at 8 wp.i. stimulated with either ESAT-6 1-15 or TB10.4 4-11 peptides or left untreated are shown. i Dot plots showing the IFN-γ secretion by lung CD8 T cells from Vhl cKO and WT mice 8 weeks after M. tuberculosis infection. j , k The frequency of Ki-67 + , tetramer-binding and total CD4 ( j ) and CD8 ( k ) T cells from lung of Vhl cKO ( n = 5) and WT mice ( n = 5) 8 w.p.i. l The fraction of lung Annexin V + CD4 and CD8 T cells from Vhl cKO ( n = 5) and WT ( n = 6) mice at 8 weeks after M. tuberculosis infection is shown. m , n The percentage of Foxp3 + CD4 T cells in the lungs ( m ) and spleens ( n ) of Vhl cKO and WT mice at 0 and 8 w.p.i. ( Vhl cKO n = 5, WT n = 4) is depicted (lungs 0 w.p.i. WT n = 4, Vhl cKO n = 4; 8 w.p.i. WT n = 5 Vhl cKO n = 8; spleens 0 w.p.i. n = 4, Vhl cKO n = 4; 8 w.p.i WT n = 4, Vhl cKO n = 5). Each symbol represents one mouse, and the data are presented as the mean ± s.e.m. The p values were calculated using a two-tailed unpaired t test with Welch’s correction and FDR adjustment for multiple comparisons. Source data are provided as a Source Data file. Full size image M. tuberculosis TB10.4 4-11 tetramer binding CD8 T cells were reduced in lungs from Vhl cKO infected mice (Fig. 2d, e ), while levels of TB10.4 tetramer binding CD8 T cells in the lungs from M. tuberculosis -infected Hif1a cKO and WT mice were similar (Fig. 2f ). In line with this observation, the fractions of IFN-γ secreting CD4 and CD8 T cells from the lungs from M. tuberculosis -infected Vhl cKO mice, stimulated respectively with ESAT-6 1-20 or TB10.4 4-11 peptides were low when comparing to those of WT cells (Fig. 2g–i ). T cells proliferate in the lung during the infection with M. tuberculosis [20] . We observed during M. tuberculosis infection, that lung Vhl cKO CD4 T cells proliferated less when compared to WT controls as measured by the expression of Ki-67 proliferation marker (Fig. 2j ). The frequency of Ki-67 expressing TB10.4 tetramer-binding CD8 T cells in lungs from M. tuberculosis- infected Vhl cKO was also lower than those the from the WT mice (Fig. 2k ). The frequency of apoptotic, Annexin V + CD4 and CD8 T cells was high in lungs from M. tuberculosis -infected Vhl cKO mice (Fig. 2l ). We investigated if increased regulatory T cells (Tregs) could account for the impaired proliferation of CD4 and CD8 T cells of Vhl cKO mice and for the enhanced susceptibility of Vhl cKO mice to M. tuberculosis infection. We found that the frequency of CD25 + Foxp3 + CD4 T cells in lungs and spleens from M. tuberculosis -infected was similar (Fig. 2m, n ). Increased expression of inhibitory receptors in T cells from Vhl cKO mice infected with M. tuberculosis Then, the impact of VHL and HIF-1 expression in T cell differentiation in the lung of M. tuberculosis infected mice was studied. We observed a preferential increase of effector memory T cells (T EM ) in lungs of WT mice infected with M. tuberculosis (Supplementary Fig. 2a–d ). Lower frequencies of CD4 but not CD8 T EM in lungs from Vhl cKO and WT M. tuberculosis -infected mice were found (Supplementary Fig. 2a, b ). Vhl cKO mice showed a high frequency of CD44 + CD62L + central memory CD8T cells (T CM ) in lungs before and during infection, while CD4 T CM were only increased in Vhl cKO at 8 weeks after infection (Fig. 3a–c ). The frequency of TB10.4 tetramer-binding within CD8 T CM cells in lungs from WT and Vhl cKO M. tuberculosis- infected mice was lower than that of TB10.4 + CD8 T EM cells (Fig. 3d ). The percentage of TB10.4 + CD8 T CM in the lungs of M. tuberculosis infected Vhl cKO and WT mice was similar. Instead, the fraction of tetramer TB10.4-binding T EM cells was lower in the lungs of Vhl cKO M. tuberculosis -infected mice as compared to WT controls (Fig. 3d ). Similar percentages of CD4 and CD8 T CM and T EM from Hif1a cKO and WT mice infected with M. tuberculosis were determined (Fig. 3e, f and Supplementary Fig. 2c, d ). Fig. 3: Decreased expression of differentiation markers and enhanced levels of inhibitory receptors in Vhl cKO T cells during M. tuberculosis infection. a – c The frequency of lung CD4 ( a ) and CD8 ( b ) T CM (CD44 + CD62L + ) from Vhl cKO ( n = 4, 5, 6, 7) and WT ( Vhl cKO ; WT n = 4, 5, 5 and 7 mice at 0, 4, 6, and 8 weeks after M. tuberculosis infection are shown. c Dot plot of CD44 and CD62L in lung CD8 T cells from Vhl cKO and WT mice 8 weeks after infection. d The frequencies of tetramer TB10.4-binding pulmonary CD8 T CM and T EM cells from Vhl cKO ( n = 6) and WT ( n = 7) mice 8 weeks after M. tuberculosis infection are depicted. e , f The fraction of pulmonary CD4 ( e ) and CD8 ( f ) T CM from Hif1a cKO and WT mice at 0 ( n = 4 per group) and 8 ( n = 5 per group) weeks after M. tuberculosis infection are depicted. g – m Dot plots ( g ) and frequency of KLRG1 + and PD-1 + CD44 + CD4 ( h , j ) and CD8 ( i , l ) T cells in the lungs of Vhl cKO and WT mice at 4 and 8 weeks after M. tuberculosis infection. The MFI of PD-1 in CD4 ( k ) and CD8 T ( m ) cells in the lungs of Vhl cKO and WT mice is also shown ( h – m ; n = 5 and 4 mice per group at 4 and 8 weeks after infection). n , o The fractions of CTLA-4 + CD4 ( n ) and CD8 ( o ) T cells in the lungs of mice before ( n = 3) and 8 weeks ( n = 4 mice per group) after infection are depicted. p – r Dot plots ( p ) and frequencies of CXCR3+ ( q ) and CX3CR1+ ( r ) CD4 and CD8 T cells in the lungs of Vhl cKO and WT mice ( n = 4 per group) 7 weeks after M. tuberculosis infection. s , t The frequency of lung parenchymal (i.v. CD45.2 negative) total ( s ) and tetramer binding ( t ) CD4 and CD8 T cells in the lungs of WT and Vhl cKO mice ( n = 5 per group) 8 weeks after infection with M. tuberculosis are shown. Each symbol represents one mouse, and the data are presented as the mean ± s.e.m. The p values were calculated using a two-tailed unpaired t test with Welch’s correction and FDR approach for multiple comparison. Source data are provided as a Source Data file. Full size image PD-1 + T cells display proliferative and protective capacity and residence in the lung parenchyma after M. tuberculosis infection, while KLRG1 is expressed in short-lived terminally differentiated effector cells [21] , [22] , [23] .We found that the cell frequency and the expression levels of KLRG1 were diminished in Vhl cKO CD4 and CD8 T cells as compared to WT controls (Fig. 3g–i , Supplementary Fig. 2e, f ). While the frequency of PD-1 + CD4 and CD8 T cells in lungs from M. tuberculosis -infected Vhl cKO and WT mice was similar, the expression levels of PD-1 were higher in pulmonary Vhl cKO CD4 and CD8 T cells from M. tuberculosis -infected mice (Fig. 3j–m and Supplementary Fig. 2g, h ). The expression of the inhibitory receptor CTLA-4 increased in CD4 (but not CD8) T cells after M. tuberculosis infection. The percentage of lung CD4 and CD8 T cells expressing CTLA-4 was higher in Vhl cKO infected mice when comparing with WT controls (Fig. 3n, o ). The T cell chemokine receptor expression pattern determines the ability to migrate into the lungs to protect against M. tuberculosis infection. Less-differentiated T cells that express CXCR3 can migrate into the lungs and suppress the growth of M. tuberculosis [21] , [24] . In contrast, T cells that express high levels of CX3CR1 poorly migrate out of the blood vessels [25] , [26] . We found reduced frequencies of both CXCR3 + and CX3CR1 + CD4 T cells from lungs of Vhl cKO mice 8 weeks after infection with M. tuberculosis when compared to those of WT controls (Fig. 3p–r ), while the fractions of CXCR3 + and CX3CR1 + CD8 T cells in lungs from Vhl cKO and WT M. tuberculosis infected mice were similar (Fig. 3q, r ). In contrast, the frequency of tetramer TB10.4 + CXCR3 + CD8 T cells in Vhl cKO was lower than WT controls (Supplementary Fig. 2i ). To determine if vascular localization of CD4 and CD8 T cells in M. tuberculosis -infected Vhl cKO mice was impaired, intravascular labeling with anti-CD45.2 mABs was performed. We found similar frequencies of extravascular (CD45.2 neg) CD4 and CD8 T cells in the lungs of M. tuberculosis -infected WT and Vhl cKO mice (Fig. 3s ), although the frequency of Vhl cKO extravascular tetramer TB10.4 + T cells was low (Fig. 3t ). More than 80% of CXCR3 + or PD-1 + T cells located in the parenchyma (Supplementary Fig. 2j, k, m ). Instead, 10% of CX3CR1 + and 20% of KLRG1 + CD4 or CD8 T cells were in the lung parenchyma of WT mice (Supplementary Fig. 2l, n, o ). The frequencies of PD-1 + , CXCR3 + , CX3CR1 + or KLRG1 + T cells that locate in the lung parenchyma of WT and Vhl cKO mice were similar (Supplementary Fig. 2k–m, o ). Altogether, during the M. tuberculosis infection of Vhl cKO mice, lung CD4 T cells showed decreased KLRG1, CXCR3, CX3CR1 and increased PD-1 and CTLA-4 levels. Some of these deviations were also observed in mutant CD8 T cells. VHL promotes proliferative and effector gene expression programs in CD4 T cells from M. tuberculosis -infected mice We then compared the global mRNA expression in sorted lung CD4 T cells from Vhl cKO and WT mice 8 weeks after infection with M. tuberculosis . We found that 3524 genes were upregulated and 3086 downregulated in Vhl deficient vs WT CD4 T cells (Fig. 4a and Supplementary Fig. 3a ). Heatmaps and unsupervised PCA analysis showed a differential clustering of WT and Vhl cKO CD4 T cells (Fig. 4b, c ). Genes involved in inhibition of T cells responses, glycolysis, and prolyl hydroxylases were among the 25 utmost differentially expressed in Vhl cKO CD4 T cells (Fig. 4a ). The gene hallmark analysis showed that hypoxia, angiogenesis, glycolysis pathways were increased in Vhl cKO CD4 T cells (Fig. 4d ), while DNA replication and metabolism, oxidative phosphorylation, MYC, E2F pathways were lower (Fig. 4e ). Within the HIF-1 pathway, glycolytic, oxygen sensing, angiogenesis related genes genes and the glucose receptor Slc2a1 were increased in Vhl cKO CD4 T cells (Fig. 4f ). The WT CD4 T cells were enriched in genes involved in lymphocyte differentiation and chemokine responses (Supplementary Fig. 3b, d ), while several transcripts involved T cell exhaustion or disfunction were increased in Vhl cKO CD4 T cells (Fig. 4g ). Fig. 4: VHL expression in lung CD4 T cells from M. tuberculosis -infected mice controls proliferation and effector responses. RNA seq was performed in Vhl cKO ( n = 6) and WT ( n = 5) CD4 T cells isolated from the lungs of M. tuberculosis -infected mice. a MA plot in which each point represents a gene. The plot illustrates the change of expression ( y axis, log 2 fold change) and the average transcript abundance over all samples ( x axis, log 2 counts per million). Colors indicate the significantly upregulated (in red) or down-regulated (in light blue) in Vhl cKO as compared to WT CD4 T cells. The top 25 most significant genes are indicated by their gene symbols. b In the heat map the log 2 counts for each gene (row) is standardized to mean = 0, and the differences with the mean depicted. c Umap dimensionality reduction plots from non-supervised samples based on the normalized gene counts after filtering the low expressed genes. There are 2 outliers in the Vhl cKO CD4 T cell group, probably explained by their lower sample weight. d , e The log 10 p value of the enrichment of hallmark gene sets in the transcriptome of Vhl cKO ( d ) and WT ( e ) CD4 T cells was compared using the MSigDB databases. f – h The heat maps of selected RNA-seq data showing: HIF-pathway-specific genes ( f ), genes involved in T cell exhaustion or dysfunction ( g ), and MYC-regulated transcripts ( h ). Data were normalized by subtracting the log 2 transformed values to the mean log 2 value for all samples for each gene. i , j Lung cell suspensions were labeled with mitochondrial-selective MitoTracker Green to assess mitochondrial mass and Mito Tracker Red to measure mitochondrial ROS. The MFI of Mito Tracker green, to assess mitochondrial mass ( i ), and Mito SOX Red, to assess mitochondrial ROS, ( j ) labeled live CD4 and CD8 T cells from the lung of Vhl cKO and WT mice ( n = 6 per group) 8 weeks after infection with M. tuberculosis are shown. i , j Each symbol represents one mouse, and the data are presented as the mean ± s.e.m. d – j The p values were calculated using a two-tailed unpaired t test with Welch’s correction ( k , m ) and FDR adjustment for multiple comparisons ( d – h ). Source data are provided as a Source Data file. Full size image Mxi1 transcripts encoding the MAX-interactor 1, a HIF-target and negative regulator of MYC expression and activity [27] was upregulated in Vhl cKO CD4 T cells. In line with a negative regulation of MYC activity, the cell cycle inhibitors Cdkn1a (p21) and Cdkn1b (p27) which are repressed by MYC [28] were increased and the cyclin dependent kinase Cdk1 transcripts were diminished in Vhl cKO CD4 T cells (Fig. 4h ). MYC and HIF-1 regulate the expression of numerous genes involved in mitochondrial biogenesis, including genes that control transcription and translation such as the mitochondrial DNA-directed RNA polymerase ( Polrmt ), and the transcription factor A mitochondrial ( Tfam ) [29] , which were found to be reduced in Vhl cKO CD4 T cells from M. tuberculosis -infected mice (Fig. 4h ). Moreover, the HIF-1 target Bnip3 and Bnip3l , coding for molecules that promote autophagy and mitophagy were increased in Vhl cKO CD4 T cells (Fig. 4h and Supplementary Fig. 3c, e ). Since metabolic pathways were widely regulated in Vhl cKO CD4 T cells during M. tuberculosis infection, we measured the mitochondrial bioenergetic profiles of lung T cells during infection with M. tuberculosis . We found that the mitochondrial mass was reduced in Vhl cKO CD4 T cells from infected mice (Fig. 4i ). Moreover, levels of mitochondrial ROS were also decreased in Vhl cKO CD4 and CD8 T cells from infected mice as compared to controls (Fig. 4j ). VHL expression is required for TCR activation of CD4 T cells Results obtained above suggested that VHL expression in CD4 T cells was critical for DNA synthesis, cell cycle progression and MYC activity. To further explore the mechanisms involved, the responses of naïve Vhl cKO CD4 T cells to T cell receptor stimulation in vitro were studied. The CD4 T cell activation increased the levels of HIF-1α in both WT and Vhl- mutant CD4 T cells. Sorted Vhl cKO CD4 T cells showed, as expected, higher levels of HIF-1α when compared to WT controls before and after TCR stimulation (Fig. 5a ). In line with this, the levels of the HIF-1 regulated transcripts Vegfa and Ldha were increased in Vhl cKO CD4 T cells before and after TCR stimulation (Supplementary Fig. 4a, b ). Fig. 5: VHL expression is required for TCR activation of CD4 T cells. a Naïve CD4 T cells were enriched by negative selection from Vhl cKO and WT spleens and stimulated with anti-CD3/CD28. Cell lysates were analysed by Western blot before and after TCR stimulation using anti-HIF-1α and anti-β-actin antibodies. One of three independent similar experiments is shown. b – d The mean % of S-phase ( b ) and G2/M ( c ) CD4 T cells and representative histograms ( d ) of the cellular DNA content after propidium iodide staining of Vhl cKO and WT CD4 T cells at different times after anti-CD3/CD28 stimulation are shown. e Cell lysates from Vhl cKO and WT CD4 T cells were analysed by immunoblot after anti-CD3/CD28 stimulation using anti-MYC or anti-β-actin antibodies. One representative of two independent experiments is shown. f Total RNA was extracted from Vhl cKO and WT CD4T cells at different times points after anti-CD3/CD28 stimulation. Cmyc mRNA titer was normalized to Hprt mRNA levels in the same samples. The Cmyc mRNA fold increase levels are depicted. g , h The frequency ( h ) and expression level ( g ) of CD71 in Vhl cKO and WT CD4T cells are shown. i The fold change levels of cd71 mRNA in Vhl cKO and WT CD4 T cells was determined by real time-PCR. j – m Representative histograms and the MFI of the TCR-β ( j , k ) and CD3 ( l , m ) expression in Vhl cKO and WT CD4 T cells are shown. Each symbol represents one independent sample, and the data are presented as the mean ± SEM. n = 3 ( b , c , f – i ), and n = 4 ( k , m ). p -values were calculated using a two-way ANOVA ( b , c ) or a two-tailed unpaired t test with Welch’s correction and a FDR adjustment ( f – i , k , m ). Source data are provided as a Source Data file. Full size image The in vitro cell cycle profile of mutant and control CD4 T cells was compared. The percentage of Vhl cKO CD4 T cells in S phase was markedly reduced when compared to that of WT controls already 16 h after anti-CD3/CD28 stimulation (Fig. 5b, d ). A large proportion of Vhl cKO CD4 T cells were in the G2/M phase compared to controls (Fig. 5c, d ). Since the oncoprotein/transcription factor MYC supports cell cycle progression, the protein expression of MYC in Vhl cKO and WT CD4 T cells was measured. MYC was rapidly induced in WT and Vhl cKO CD4 T cells after TCR stimulation, but the level of MYC in Vhl cKO CD4 T cells after TCR-stimulation was attenuated (Fig. 5e ). The Myc mRNA levels in WT and Vhl cKO CD4 T cells before or after TCR stimulation were similar, suggesting that the reduction in MYC protein level in Vhl cKO CD4 T cells is regulated at the post-transcriptional level (Fig. 5f ). The anti-CD3/CD28 triggering of WT CD4 T cells increased the expression of CD71, the transferrin receptor, a downstream target of MYC. The expression level and the frequency of CD71 expressing Vhl cKO CD4 T cells was low when compared with WT controls (Fig. 5g, h ). The accumulation of Cd71 mRNA was also reduced in anti-CD3/CD28-stimulated Vhl cKO CD4 T cells when compared to controls (Fig. 5i ). The titers of Mxi1 mRNA, coding for a MYC-negative regulator, and of Cdkn1a mRNA was higher in Vhl cKO than in WT CD4 T cells (Supplementary Fig. 4c, d ). We also found a reduced level of expression of the TCR-β, CD3ε and CD4 receptors in Vhl cKO CD4 T cells compared to that in WT cells (Fig. 5j–m and Supplementary Fig. 4e, f ), indicating that differences in the expression of diverse components of the TCR complex prior to stimulation can account for the diminished activation of Vhl cKO CD4 T cells. VHL promotes proliferation of CD4 T cells after TCR stimulation MYC drives both cell growth and proliferation. We observed that the frequency of Vhl cKO CD4 T cells after anti-CD3/CD28 stimulation of splenocytes was low, resembling changes in T cell frequencies during infection in vivo (Fig. 6a–c ). Instead, the frequencies of Hif1a cKO and WT T cell populations were similar (Fig. 6a–c ). The proliferation of TCR-stimulated Vhl cKO CD4T cells was impaired while that of CD8 T cells was reduced when compared to WT controls (Supplementary Fig. 5a–c ). The proliferative responses of anti-CD3/CD28-stimulated naïve Vhl cKO CD4 T cells were abolished (Fig. 6d, e ). Fig. 6: VHL promotes proliferation of CD4 T cells in response to TCR activation. a – c The % CD4 ( a ), CD8 ( b ) and DN ( c ) T cells in Vhl cKO ( n = 3), Hif1a cKO ( n = 3) and WT ( n = 6) spleen cell suspensions measured 6 days after anti-CD3/CD28 stimulation is shown. d Representative histogram of CFSE-labeled Vhl cKO and WT CD4 T cells 3 days after stimulation with anti-CD3/CD28 are shown. e The CFSE labeling was used to calculate the division index (the average number of cell division that a cell in the original population has undergone). f – h Dot plots showing the FCS/SSC of lymphocyte gated Vhl cKO and WT CD4 T cells before and 48 h after stimulation with anti-CD3/CD28 ( f ). The mean percentage of blast cells ( g ) and the FSC of blasts ( h ) 48 h after anti-CD3/CD8 stimulation are shown. i , j The percentage of CD69+ ( i ) and CD44 +  ( j ) Vhl cKO and WT CD4 T cells after anti-CD3/CD28 stimulation are depicted. k The titers of IL-2 in the culture supernatants from Vhl cKO and WT CD4 T cells before and 48 h after anti-CD3/CD28 stimulation. l , m The percentage of cells expressing CD25 ( l ) and the MFI of CD25 ( m ) on TCR-stimulated Vhl cKO and WT CD4 T cells is depicted. n The percentage of Annexin V + Vhl cKO and WT CD44 + CD4 T cells 3 days after stimulation with anti-CD3/CD28. e , g – n n = 3 independent cultures per group. o , p Rag2 −/− mice were transferred i.v. with either 2.10 6 CD4 T cells from CD45.2 Vhl cKO , CD45.1 WT or a mixed 1:1 suspension from both genotypes (10 6 cells/each). The percentages and numbers of CD4 T cells in the spleen ( o , p ) and blood ( q ) of mice 5 weeks after transfer is shown ( n = 4 mice per group). Each symbol represents one independent biological sample, and the data are presented as the mean ± SEM. p -values were analysed using two-tail unpaired t test ( e , g – n ) with FDR adjustment or one-way ANOVA with Welch’s correction ( a – c , o – q ). Source data are provided as a Source Data file. Full size image The growth response of Vhl cKO CD4 T cells after anti-CD3/CD28 stimulation was markedly reduced when compared to WT controls (Fig. 6f–h and Supplementary Fig. 5d ). T cells express CD69 and CD44 early after TCR triggering. The expression density and the frequencies of CD69 + and CD44 + CD4 T cells increased from 24 to 48 h after anti-CD3/CD28 stimulation (Fig. 6i, j and Supplementary Fig. 5e–h ). Despite the reduced growth and proliferative responses, the frequencies of CD69 and CD44 expressing Vhl cKO and WT CD4 T cells and their expression levels 24 h after anti CD3/CD28 stimulation were similar (Fig. 6i, j and Supplementary Fig. 5e–h ). Instead, 48 h after TCR stimulation the percentages of CD69 + and CD44 + Vhl cKO CD4 T cells were low compared to those of WT cells (Fig. 6i, j and Supplementary Fig. 5e, h ). The intensity of CD44 on Vhl cKO CD4 T cells, but not that of CD69, 48 h after anti-CD3/CD28 stimulation was lower when compared to WT controls (Supplementary Fig. 5e–h ). IL-2 augments T cell proliferation and survival. The accumulation of IL-2 in supernatants of anti-CD3/CD28 stimulated Vhl cKO CD4 T cells cultures was impaired (Fig. 6k ), in line with their deficient proliferative responses. The expression of CD25, the α-chain of the IL-2 receptor, was upregulated in naïve CD4 T cells after TCR activation (Fig. 6l, m ). The expression levels of CD25 were also lower in Vhl cKO CD4 T cells than in WT controls (Fig. 6l, m ). Thus, both IL-2 production and the expression of the high affinity IL-2 receptor were muted in Vhl cKO CD4 T cells after stimulation with anti-CD3/CD28. The addition of exogenous IL-2 did neither restore the proliferation, the CD44 expression nor resulted in increased cell size of TCR-stimulated Vhl cKO CD4 T cells (Supplementary Fig. 5i–k ). The frequency of Annexin V expressing TCR-triggered Vhl cKO CD4 T cells was high compared to WT controls (Fig. 6n and Supplementary Fig. 5l ). Homeostatic proliferation of T cells occurs when small numbers of T cells are adoptively transferred into immunodeficient hosts [30] . WT but not Vhl cKO CD4 T cells were detected in the blood and spleens of recipient Rag2 −/− mice single transferred or co-transferred with 2.10 6 WT or/and Vhl cKO CD4T cells (Fig. 6o-q and Supplementary Fig. 5m, n ). HIF-1 mediates the susceptibility to M. tuberculosis -infection of Vhl cKO mice To investigate whether HIF-1 overexpression mediates the increased M. tuberculosis susceptibility of Vhl cKO mice, Hif1a fl/fl Vhl fl/fl cd4 cre (Vhl Hif1a dcKO) mice were generated. Vhl Hif1a dcKO and WT mice showed similar bacterial levels in spleens and lungs 4 and 7 weeks after aerosol M. tuberculosis infection (Fig. 7a, b ). The proportion and numbers of T cells and the frequencies of CD4 and CD8 T cells in lungs of Vhl Hif1a dcKO and WT mice at 4 and 7 weeks after M. tuberculosis infection were similar (Fig. 7c, d and Supplementary Fig. 6a–d ). The percentage of ESAT-6 and TB10.4 tetramer-binding CD4 and CD8 T cells that were reduced in Vhl cKO infected compared to WT mice, were similar in WT and Vhl Hif1a dcKO mice (Fig. 7e, f ). Lungs of Vhl Hif1a dcKO and WT mice also showed similar frequencies of central and effector memory CD4 and CD8T cells at 4 and 7 weeks after infection (Fig. 7g, h and Supplementary Fig. 6e–h ). Further, the expression levels of PD-1, KLRG1, CXCR3 and CX3CR1 in CD4 T cells from WT and Vhl Hif1a dcKO mice at 4 and 7 weeks after M. tuberculosis infection were comparable (Fig. 7i–l and Supplementary Fig. 6i–l ). The fraction of PD-1-, KLRG1-, CXCR3- and CX3CR1-expressing CD8 T cells from WT and Vhl Hif1a dcKO was also similar (Fig. 7m–p , Supplementary Fig. 6m–p ). Altogether, HIF-1 stabilization mediates the susceptibility of Vhl cKO mice during infection with M. tuberculosis and the distinct phenotype of T cells of Vhl cKO during the bacterial infection. Fig. 7: HIF-1 mediates the susceptibility to M. tuberculosis -infection of Vhl cKO mice. a , b Vhl cKO, Vhl Hif1a dcKO and WT mice were sacrificed at 4 ( a ) and 7 ( b ) weeks after aerosol infection with M. tuberculosis . The log 10 CFU in lungs and spleens are depicted; ( a ) WT n = 9, Vhl Hif1a dcKO n = 8, ( b ) WT n = 6, Vhl cKO n = 6, Vhl Hif1a dcKO n = 9. c , d The frequency of CD4 ( c ) and CD8 ( d ) T cells in the lung of Vhl Hif1a dcKO , Vhl cKO and WT mice 7 weeks after M. tuberculosis infection is shown. e , f The percentage of tetramer ESAT-6-binding CD4 T cells ( e ) and TB10.4-binding CD8 T cells ( f ) in the lung of Vhl Hif1a dcKO , Vhl cKO and WT mice 7 weeks after infection are displayed. g , h The frequency of CD4 ( g ) and CD8 ( h ) T CM in the lung of Vhl cKO, Vhl Hif1a dcKO and WT mice 7 weeks after M. tuberculosis infection is shown. i – p The frequency of KLRG1 +  ( i , m ), PD-1 +  ( j , n ), CXCR3 +  ( k , o ) and CX3CR1 +  ( l , p ) CD4 and CD8 T cells in the lung of Vhl Hif1a dcKO , Vhl cKO and WT mice 7 weeks after infection with M. tuberculosis . c – p n = 5 mice per group. Each symbol represents one mouse, and the data are presented as the mean ± SEM. p -values were calculated using one-way ANOVA test with Welch’s correction for unequal SD and Dunnet’s T3 adjustment for multiple comparisons. Source data are provided as a Source Data file. Full size image HIF-1 stabilization in T cells impairs the responses to immunization with BCG Whether VHL-deficiency in T cells also regulated the responses to immunization with the attenuated M. bovis BCG was studied. Vhl cKO, Vhl Hif1a dcKO and WT mice were administered with BCG i.v. and the T cell phenotype in lungs and spleens analysed 3 weeks after immunization. The Vhl cKO mice showed lower percentage of CD4 T cells in lungs and spleens as compared to WT and Vhl Hif1a dcKO after BCG immunization, while the frequencies of the T cell populations in non-immunized mice were similar (Fig. 8a, b and Supplementary Fig. 7a ). The frequency of CD8 T cells (but not of DN T cells) was increased in the lungs (but not spleens) of Vhl cKO mice as compared to WT and Vhl Hif1a dcKO mice (Fig. 8c and Supplementary Fig. 7b ). Since ESAT-6 is not expressed by BCG, I-A b Ag85b 280-294 tetramers were used to quantify BCG-specific CD4 T cells in immunized mice. The frequency of tetramer Ag85b-binding CD4 T cells and of TB10.4-binding CD8 T cells was reduced in lungs and spleens of immunized Vhl cKO when compared with Vhl Hif1a dcKO and WT mice (Fig. 8d–g and Supplementary Fig. 7c, d ). Further, the frequencies of CD4 and especially that of CD8 T CM in lungs and spleens from immunized Vhl cKO were higher (Fig. 8h, i and Supplementary Fig. 7g, h ), whereas levels of CD4 and CD8 T EM were reduced when comparing to WT and Vhl Hif1a dcKO mice (Fig. 8j, k and Supplementary Fig. 7e, f ). The frequency of CD8 T CM in the lungs and spleens of non-immunized Vhl cKO was higher than those of WT and Vhl Hif1a dcKO mice (Fig. 8i and Supplementary Fig. 7h ). Fig. 8: HIF-1 stabilization in T cells impairs the responses to immunization with BCG. a – c The frequency of total ( a ), CD4 ( b ) and CD8 ( c ) T cell populations in lungs before and 3 weeks after i.v. immunization with BCG are depicted. d – g The percentages ( d , f ) and representative dot plots ( e , g ) of tetramer Ag85b-binding CD4 T cells ( d , e ) and TB10.4 tetramer-binding CD8 T cells ( f , g ) in the lungs of Vhl Hif1a dcKO , Vhl cKO and WT mice ( n = 5 per group) after BCG immunization are shown. The frequencies of T CM ( h , i ), T EM ( j , k ) in CD4 and CD8 T cells in lungs from Vhl Hif1a dcKO , Vhl cKO and WT mice at 0 or 3 weeks after BCG immunization are depicted. l The percentage of lung CD49d + CD8 T CM before and after BCG immunization of WT and Vhl cKO mice are shown. The frequencies of KLRG1 +  ( m , n ) and CX3CR1 +  ( o , p ) in CD4 and CD8 T cells in lungs from Vhl Hif1a dcKO , Vhl cKO and WT mice at 0 or 3 weeks after BCG immunization are depicted. q The fraction of CTLA-4 + CD4 and CD8 T cells in the lung of BCG immunized mice are shown. Each symbol represents one mouse, and the data are presented as the mean ± SEM ( a – k , m – p ) before immunization n = 3 per mice per group, after immunization n = 5 per group; l before n = 4 per group, after immunization n = 5 per group; q n = 5 per group. p -values were calculated using 2-way ANOVA test, with Sidak adjustment for multiple comparisons. Source data are provided as a Source Data file. Full size image CD8 T cells may exhibit a memory phenotype without overt immunization or infection. These cells, unlike true memory T cells that develop in response to foreign antigen, express only low levels of CD49d and are termed virtual memory T (T VM ) cells [31] , [32] , [33] . The CD44 + CD62L + CD8 T cells in spleens and lungs from non-immunized mice expressed low levels of CD49d suggesting these are T VM cells (Fig. 8l and Supplementary Fig. 7i ). The frequency of CD49d expressing WT CD8T CM increased after immunization while levels in remained low in the Vhl cKO CD8T cells (Fig. 8l ). The fractions of KLRG1 + and CX3CR1 + CD4 and CD8 T cells in lungs and spleens from Vhl cKO mice were lower than those in WT and Vhl Hif1a dcKO mice (Fig. 8m–p and Supplementary Fig. 7j–m ). Lower percentages of CXCR3 + CD4, but not CD8 T cells, were also recorded in the spleens (but not lungs) of Vhl cKO BCG immunized mice (Supplementary Fig. 7n, o ). Different to infected mice, PD-1 levels were not increased in pulmonary or splenic Vhl cKO T cells as compared to those of WT or Vhl Hif1a dcKO mice (Supplementary Fig. 7p, q ). However, the frequencies of CTLA-4 + CD4 and CD8 T cells from lungs of BCG-immunized Vhl cKO mice were higher than those measured in WT controls (Fig. 8q ). We found that the BCG CFU titers in the spleens and lungs from Vhl cKO were higher than those in WT mice, indicating that either clearance or control of dissemination of BCG was impaired in Vhl cKO mice. No overt signs of clinical disease were observed during the experiment (Supplementary Fig. 7r ). Altogether, Vhl -deficiency resulted in a HIF-1 dependent reduction of the pulmonary and splenic CD4 T cells and of specific T cell responses after BCG-immunization. As observed during infection the levels of the differentiation markers CX3CR1 and KLRG1 were reduced and the expression of CTLA-4 increased in T cells from immunized Vhl cKO mice. HIF-1 stabilization impairs CD4 T cell responses in vitro We then studied whether HIF-1α overexpression accounts for the impaired TCR responses of Vhl -deficient CD4 T cells. We found that the growth response (Fig. 9a, b ), the fraction of different cell cycle phases (Fig. 9c, d ), the proliferation (Fig. 9e and Supplementary Fig. 8a ) and the CD44 expression levels (Supplementary Fig. 8b ) in WT and Vhl Hif1a dcKO CD4 T cells at different times after TCR-activation were similar. Fig. 9: HIF-1 stabilization impairs CD4 T cell responses in vitro. a , b The FSC of blasts ( a ) and the % cell size increase relative to unstimulated cells in the blast population ( b ) were depicted. c , d The % of S-phase ( c ) and G2/M ( d ) of CD4 T cells are shown. e CFSE profiles of Vhl Hif1a dcKO and WT CD4 T cells 3 days after stimulation with anti-CD3/CD28 are shown. f – m RNA-seq was performed in independent cultures of WT ( n = 4), Vhl cKO ( n = 3) and Vhl Hif1a dcKO CD4 T ( n = 4) cells before or 24 h after anti CD3/CD28 stimulation. f The Pearsson R 2 correlation matrix of the expression of all genes in each sample is shown. g Heat map of the log 2 counts for each gene standardized to the mean. h , i Volcano plots showing the log 2 fold change in gene expression ( x -axis) and p -value ( y -axis), of differentially upregulated or downregulated genes ( p ≤ 0.05 and log 2 fold change > 1) ( i ). j , k The log 10 p value of the most enriched KEEG-pathway terms in Vhl cKO vs WT ( j ) or in WT vs Vhl cKO CD4 T cells ( k ). l , m The MFI ( l ) and a representative histogram ( m ) of phospho-rpS6 on WT and mutant CD4 T cells 2 h after anti-CD3/CD28 or PMA/I stimulation are illustrated. n The frequency of IFN-γ expressing WT, Vhl cKO and Vhl Hif1a dcKO CD4 T cells 6 h after PMA/I or 72 h after anti-CD3/CD28 stimulation are shown. A group was stimulated with anti-CD3/CD28 for 65 h and then incubated for 6 h with PMA/I. a – d , l , n Each symbol represents one independent sample ( n = 3 per group), and the data are presented as the mean ± SEM. p -values were calculated using a two-tailed unpaired t test with Welch’s correction ( a – d ) and 2-way ANOVA test, with Sidak adjustment for multiple comparisons ( l , n ). Source data are provided as a Source Data file. o VHL promotes the cell cycle progression, growth responses, proliferation, IL-2 secretion and expression of activation markers of TCR-stimulated CD4 T cells, the differentiation and the protective function of T cells against M. tuberculosis infection as well as the responses to immunization by impairing HIF-1 stabilization. Full size image The transcriptome profile of WT, Vhl cKO and Vhl Hif1a dcKO CD4 T cells stimulated with anti-CD3/CD28 was then compared. The correlation analysis of the biological replicates (Fig. 9f ), the heat map (Fig. 9g ) and the principal component analysis (Supplementary Fig. 8c ) showed the segregation of the transcriptome of unstimulated WT CD4 T cells in comparison to the other groups. Within the TCR-stimulated groups the gene expression of Vhl cKO CD4 T cells differed to that of WT and Vhl Hif1a dcKO CD4 T cells that showed important similarities between them (Fig. 9f–g ). The Vhl cKO CD4 T cells expressed higher number of unique transcripts (499) and lower number of common genes as compared to either Vhl Hif1a cKO or WT CD4 T cells after anti-CD3/CD28 stimulation (Supplementary Fig. 8d ). Eight hundred thirty nine genes were increased and 1078 were reduced in WT as compared to Vhl cKO CD4 T cells after anti CD3/CD28 stimulation (Supplementary Fig. 8e ). Low numbers of differentially expressed genes were detected when comparing WT vs Vhl Hif1a dcKO CD4 T (Fig. 9h, i and Supplementary Fig. 8e ). 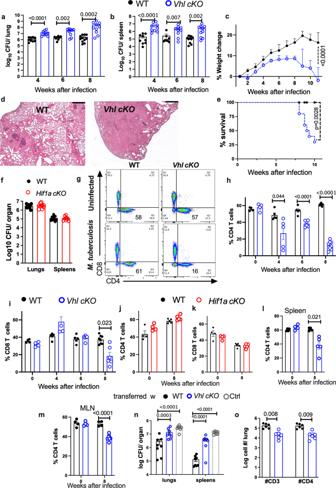Fig. 1: VHL expression in T cells is critical for the control ofM. tuberculosisinfection in mice. a,bVhl cKOand WT mice were infected via aerosol with 250M. tuberculosisand sacrificed at indicated time points after infection. The log10CFU in the lung (a) and spleen (b) of individual mice (nWT = 10, 9, 12;nVhl cKO= 9, 9, 10 mice at 4, 6 and 8 weeks post infection (w.p.i.) respectively) are represented.cThe weight change with respect to the uninfected group mean (day 0) during infection withM. tuberculosisofVhl cKOand WT mice (n= 11 per group) is depicted.dRepresentative micrographs from hematoxylin-eosin-stained paraffin lung sections fromVhl cKOand WT mice 8 w.p.i. withM. tuberculosis(bar: 400 μm).eThe cumulative mortality ofVhl cKOand WT mice (n= 9 per group) afterM. tuberculosisinfection is depicted.fThe log10CFU in the lungs and spleens ofHif1a cKO(n= 11) and WT (n= 9) mice 8 w.p.i. withM. tuberculosisare shown.g–iThe representative dot plots of CD4 and CD8 (gated on T cells) in the lungs ofVhl cKOand WT mice before and 8 w.p.i. withM. tuberculosis(g), and the frequency of CD4 (h) and CD8 (i) T cells in the lungs (WTn= 4, 4, 6, 8 andVhl cKOn= 4, 5, 6 and 8 mice at 0, 4, 6 and 8 w.p.i. respectively).j,kThe frequency of CD4 and CD8 T cells in the lungs ofHif1a cKOand WT mice before (n= 4 per group) and 8 w.p.i. (n= 5 per group) are depicted.l,mThe frequency of CD4 in spleens (l) and mediastinal lymph nodes (m) before and 8 w.p.i. withM. tuberculosisare shown (Vhl cKOn= 4, 7 and WTn= 4, 4 mice at 0 and 8 w.p.i., respectively).Rag2−/−mice were administered i.v. with either 2.106Vhl cKOor WT CD4 T cells (n= 6) or left untreated 3 days afterM. tuberculosisinfection. The log10CFU in the lungs and spleens (n) (n= 8 animals per group) and number of CD4 T cells (o) in lungs (n= 6 mice per group) 4 w.p.i. Each symbol represents one mouse, and the data are presented as the mean ± s.e.m. Thep-values were calculated using either a two-tailed unpairedttest with Welch’s correction for no homoscedasticity and FDR approach for multiple comparison (a,b,f,h–m,o), a one-way ANOVA with Welch’s correction (n), a 2-way ANOVA with Sidak’s multiple comparison test (c), or a χ2test (e). Source data are provided as a Source Data file. Among the 45 highest ranked differentially expressed transcripts in Vhl cKO vs WT CD4 T cells, 11 play a role in glycolysis, 8 are immune regulators, 5 are involved in oxygen sensing and 4 are inhibitors of proliferation (Supplementary Table 1 ). The KEEG pathway enrichment analysis showed that genes in the HIF-1 signaling and carbon metabolism pathways were enriched in TCR stimulated Vhl cKO as compared WT CD4 T cells, while genes involved in the positive regulation of cell cycle, mitosis and Rho GTPase activation were increased in WT as compared to Vhl cKO CD4 T cells (Fig. 9j, k ). Upregulated genes in the HIF-1 pathway play a role in glycolysis, oxygen sensing, mitochondrial autophagy, cell cycle inhibition, angiogenesis and immune responses (Supplementary Fig. 8f ). The GO analysis identified T cell activation, cytokine production, response to oxygen processes and dioxygenases enriched in anti-CD3/CD28 stimulated Vhl cKO as compared to WT CD4 T cells (Supplementary Fig. 8g, i ). Genes involved in cell cycle/mitosis were increased in WT vs Vhl cKO CD4 T cells (Supplementary Fig. 8h, j ). The phosphorylation of the ribosomal protein 6 (rpS6) is a key component of the translational machinery in eukaryotic cells and a point of convergence for multiple signaling pathways downstream of the TCR [34] . While the frequency of WT, Vhl cKO and Vhl Hif1a dcKO CD4 T cells expressing phospho-rpS6 after anti-CD3/CD28 stimulation was similar the expression levels were reduced in Vhl cKO as compared to WT and Vhl Hif1a dcKO CD4 T cells (Fig. 9l, m and Supplementary Fig. 8k ). Instead, the levels of phospho-rpS6 expression in WT and mutant CD4 T cells after PMA/I stimulation were similar (Fig. 9l ), suggesting that PMA/I activation bypasses the HIF-1-mediated inhibition of a TCR proximal signaling. In line with this, the frequency of IFN-γ-secreting Vhl cKO CD4 T cells after anti-CD3/CD28 stimulation was lower than those from WT or Vhl Hif1a dcKO CD4 T cells, while the frequency of IFN-γ secreting Vhl cKO , Vhl Hif1a dcKO and WT CD4 T cells stimulated with PMA/I was similar (Fig. 9n ), also indicating that T cell activation in response to PMA/I is not impaired in Vhl cKO CD4 T cells. In agreement with the suggestion that TCR- activation is impaired upon Vhl-loss, the levels of CD44, CD69 and CD25 levels as well as the proliferative responses of Vhl cKO CD4 T cells were diminished in response to stimulation with the Staphylococcal enterotoxin B superantigen (SEB) (Supplementary fig. 9a–k ). Instead, the fraction of CD44, CD69 and CD25 expressing WT and Vhl cKO T cells stimulated with PMA/I were similar (Supplementary fig. 9l–n ). Here, we report that stabilization of HIF-1 in T cells dramatically increased susceptibility to infection with M. tuberculosis that associated with a defective accumulation of mycobacteria-specific T cells in the lungs, and the lack of ability of Vhl cKO CD4 T cells to confer resistance against infection upon transfer. M. tuberculosis as many other pathogenic bacteria and viruses have evolved a strategy of persistence to optimize transmission [35] . A HIF-1 control of T cell functions and differentiation was not found to be an adaptation to allow mycobacterial evasion and chronic infection, since, after immunization with BCG, Vhl cKO mice also showed reduced accumulation of mycobacterial-specific CD4 and CD8 T cells, diminished CD4 T cell frequencies and low levels of the differentiation markers KLRG1 and CX3CR1 in lung and spleen CD4 and CD8 T cells and high levels of the inhibitor receptor CTLA-4. Our in vivo and in vitro data disclosed that after TCR-stimulation, VHL-deficient CD4 T cells showed decreased growth response, altered cell cycle progression, reduced proliferation and increased expression of apoptotic markers, responses that were regulated by the transcription factor MYC. MYC, like HIF-1, has pleiotropic effects on metabolism, proliferation, and cell growth of different cell populations including T cells. In T cells, MYC is regulated by TCR and IL-2 signaling and supports T cell differentiation [36] . MYC also regulates IL-2 responses but adding IL-2 to Vhl cKO CD4 T cells did not restore the proliferative responses after TCR stimulation, suggesting that the defect in IL-2 generation alone is not solely responsible for the activation defects of Vhl cKO CD4 T cells. Studies of hypoxia-induced cell cycle arrest have demonstrated that HIF-1 counteracts the effects of MYC on proliferation, although HIF-1 and MYC can also have synergistic effects on angiogenesis and metabolic responses [15] , [37] . The overexpression of HIF-1 has been shown to displace MYC from its DNA binding sites, leading de-repression of the genes coding for cyclin dependent kinases (CDK) inhibitors p21 and p27 [37] , [38] . HIF-1 has been also shown to mediate regulation of MYC via the induction of the MYC-antagonist MXI-1 [15] , [39] and the promotion of the proteasome-dependent degradation of MYC [15] . Others have shown that HIF-1α can directly interact with Mcm replication proteins to regulate cell cycle progression [40] . Accordingly, mxi1, cdnk1a and cdkn1b transcripts were increased in Vhl cKO CD4 T cells in the lungs of M. tuberculosis -infected mice, where genes involved in proliferation, cell cycle progression and mitochondrial activity were downregulated. We suggest that Vhl-deficiency required for early molecular events after TCR-mediated activation after anti-CD3/CD28 or SEB-stimulation. Bypassing direct TCR signaling with PMA/ionomycin normalized the early Vhl cKO CD4 T cell responses. Homeostatic proliferation of CD4 and CD8 T cells has been shown to require the contact with self-MHC class II and I molecules, respectively [41] , [42] , [43] . Thus, the deficient Vhl cKO CD4 T cells reconstitution in blood and spleen from Rag2 − /− lymphopenic mice also supports a TCR-signaling defect of the mutant cells. The loss of HIF-1 in CD4 T cells has been shown to compromise help during antibody responses, and the ability of both CD4 and CD8 T cells to produce IFN-γ [44] HIF-1 has also been shown to enhance Th17 as well as IFN-γ secretion and attenuate the development of Treg cells [45] , [46] , [47] , [48] . The deficiency of VHL in CD8 T cells resulted in improved control of persistent viral infection and neoplastic growth in a HIF-dependent manner [16] , [18] . VHL deficiency resulted in a sustained CD8 T cell effector phenotype and T cell activation [16] , [18] , without impairing the formation of memory cells [49] . In line with this, the loss of PHD proteins expanded T H 1 responses, limited Treg induction, and enhanced CD8 T cell effector functions [17] . In contrast to these observations, hypoxia has been shown to inhibit the proliferation of numerous cell types in a HIF-1-dependent manner [38] , [50] , and overexpression of HIF-1 or HIF-2 alone was sufficient to induce cell cycle arrest in normoxic conditions [51] . T cells activated under hypoxic conditions showed reduced proliferation, impaired effector functions and increased cell death [52] , [53] , [54] , [55] . The inhibition of glycolysis (and HIF-1 expression) enhanced memory-like CD8 T cells and artificially enforcing glycolytic metabolism restricted the generation of memory CD8 T cells [56] . In line with our results, VHL expression in mature T cells has been shown to promote follicular helper T cell and T H 17 differentiation [48] , [57] . The expression of inhibitory receptors CTLA-4, PD-1, Cd73, Nr4a2 and Nr4a3 in Vhl cKO CD4 T cells was increased while transcription factors and molecules involved in T cell differentiation (T-bet, eomes, CX3CR1 and KLRG1) were downregulated in Vhl cKO CD4 T cells, during M. tuberculosis infection. A reduction of CD4, but not of CD8 T cells frequencies, a high expression of inhibitory molecules and low levels of chemokine receptors were observed in the lungs and spleens of M. tuberculosis -infected or immunized Vhl cKO mice. Lungs and spleens from Vhl cKO infected, immunized and control mice, showed a higher frequency of CD44 + CD62L + CD8 T cells than WT mice. In non-immunized mice these cells lacked CD49d expression suggesting that they are T VM cells, antigen-naïve T cells that bear markers of homeostatic expansion [30] , [58] . After infection, the lung Vhl cKO CD8 T CM showed low levels of TB10.4 tetramer positive cells as well as low CD49d expression. In normal mice T VM have been shown to comprise 5-20% CD8 T cells, and have been shown to preferentially differentiate into CD8 T CM [30] , [58] . Virtual memory CD8 T cells have been shown to display low IFN-γ responses but could productively contribute to antigen-specific responses against invading viruses [59] , [60] and bacteria [61] , and can account for the discrepancies indicated above. The fraction of Vhl cKO CD44 + CD62L + CD4 T cells in lungs or spleens was in comparison low. VHL mediates the proteasomal degradation of both HIF-1α and HIF-2α subunits. HIF-2 has both distinct and overlapping biological roles with HIF-1. HIF-1 has been shown to induce apoptotic pathways and drive the expression of genes that are involved in the glycolytic pathway, whereas HIF-2 preferentially promotes growth and angiogenesis [30] , [62] . Whereas HIF-1 is ubiquitously expressed, the expression of HIF2 is mainly restricted to endothelial, lung, renal and hepatic cells [63] . The ablation of the Vhl gene increased the expression of HIF-2 in CD8 T cells [16] and HIF-2 deletion in T regs has been shown to impair their suppressive function (through the increase of HIF-1 levels) [64] . Ectopic expression of HIF-2α, but not HIF-1α increased cytotoxic, differentiation and cytolytic function against tumor targets of CD8 T cells [65] . VHL has also HIF-independent functions, regulating apoptosis, cell senescence and transcription among other programs [66] , [67] . Our data indicates that impaired T cell-mediated protection against M. tuberculosis in Vhl cKO mice was due to stabilization of HIF-1. Redundant gene regulation by HIF-2 or the HIF-independent functions of VHL did not account for the dysfunctional CD4 T cells in Vhl cKO observed. Moreover, the altered metabolic responses in Vhl cKO CD4 T cells were restored when in Vhl Hif1a dcKO mice. Thus, we showed HIF-1 play impairs CD4 T cell activation and differentiation leading to an increase susceptibility to infection with M. tuberculosis and impaired responses to vaccination (Fig. 9o ). While this may have ample consequences in diverse microbial insults, we suggest that the hypoxic environment of the TB granuloma, by impairing local CD4 T cell functions [68] , may contribute to bacterial survival and chronicity of infection. Mice The animals were housed according to directives and guidelines of the Swedish Board of Agriculture, the Swedish Animal Protection Agency, and the Karolinska Institutet (djurskyddslagen 1988:534; djurskyddsförordningen 1988:539; djurskyddsmyndigheten DFS 2004:4). The study was performed under approval of the Stockholm North Ethical Committee on Animal Experiments permit number 1374-2020 and N128/16. Mice were housed at the Comparative Medicine Biomedicum and the Astrid Fagræus Laboratories, Karolinska Institutet, Stockholm, under specific pathogen-free conditions. All mice in this study were between 8–15 week/old. Mice were maintained in a specific pathogen free unit on a 12 h light/12 h dark cycle. Room temperature was maintained at 25 °C. The humidity level was controlled between 40–60%. Mice containing loxP-flanked Hif1a and Vhl alleles have been previously described [69] , [70] . For a T-cell-specific deletion, these were bred with transgenic mice containing Cre -recombinase gene driven by the distal promoter of the lymphocyte protein tyrosine kinase ( dlck cre ) [71] or under the CD4 promoter ( cd4 cre ) [72] both resulting in cre expression during the DP stage thymocyte development. Hif1a fl/fl or Vhl fl/fl littermates were used as controls. Vhl fl/fl and hif1 fl/fl cd4 cre mice were also crossed to generate mice lacking both Hif1a and Vhl genes in T cells. The C57BL/6 (Ly5.1 B6) congenic strain carrying the differential pan leukocyte marker CD45.1 and T and B-cell deficient Rag2 −/− mice with a C57Bl/6 background were used in T-cell co-transfer mice studies. Infection and infectivity assay M. tuberculosis Harlingen and BCG Montreal were grown in Middlebrook 7H9 (Difco, Detroit, MI) supplemented with albumin, dextrose, catalase and, for BCG cultures, 50 µg/ml hygromycin (Sigma, St. Louis, MO). Mice were infected with 250 M. tuberculosis Harlingen strain by aerosol using a nose-only exposure unit (In-tox Products, Moriarty, NM), or immunized i.v. with 10 7 BCG. To determine viable numbers of M. tuberculosis and BCG CFUs at different time-points post-infection, the right lung of each mouse was homogenized in PBS with 0.05% Tween 80. Bacteria were quantified on Middlebrook 7H11 agar containing 10% enrichment of oleic acid, albumin, dextrose, catalase, 5 µg of amphotericin B per ml and 8 μg/ml polymyxin B grown for 3 weeks at 37 °C. Naïve CD4 T cell isolation and activation in vitro Single cell suspensions were obtained from spleens of mice by mechanical disruption, filtering over a 70 μm nylon cell strainer and lysis of erythrocytes. Label-free naïve CD4 + CD44 − T cells were further isolated by negative selection using magnetic beads (MACS, Miltenyi Biotec, Germany). After counting, splenocytes were resuspended in PBS with 0.5% bovine serum albumin (BSA) and 2 mM EDTA, incubated with biotin-conjugated anti-CD44 microbeads and applied through a separation column under a magnetic field. Selected cells were then resuspended in RPMI-1640 media supplemented with 5% FCS and penicillin/streptomycin stimulated in vitro with either plate-bound anti-CD3 antibody (145-2C11, Invitrogen, Waltham, MS) and soluble anti-CD28 antibody (37.51, BD, Franklin Lakes, NJ), with 50 ng/ml phorbol myristate acetate (PMA) and 2 μg/ml ionomycin (Sigma, StLouis, MO), or with 20 μg/ml Staphylococcal enterotoxin B (SEB) (Sigma) and cultured at CO 2 incubator at 37 °C and 5% CO 2 . Flow cytometry Surface markers Lungs were removed, mechanically minced into small pieces and digested with 3 mg/ml Collagenase D and 30 μg/ml DNase I for 1 h at 37 o C, and single-cell suspensions prepared by filtering lung tissue through 70 µm nylon cell strainers. To enrich the suspension in lymphocytes, cells were loaded into an isotonic 40–70% Percoll density gradient and centrifuged for 30 min at room temperature. Cells in the gradient interphase were collected and washed before further culturing/labeling. Mediastinal lymph node cell suspensions were obtained after mechanical disruption of the followed by filtering over a 70-µm nylon mesh. Single spleen cell suspensions were obtained by mechanical disruption, lysis of erythrocytes and straining over a 70-µm nylon mesh. Cell suspensions were incubated with live/dead stain (LIVE/DEAD™ Fixable Yellow Dead Cell Stain, Invitrogen). 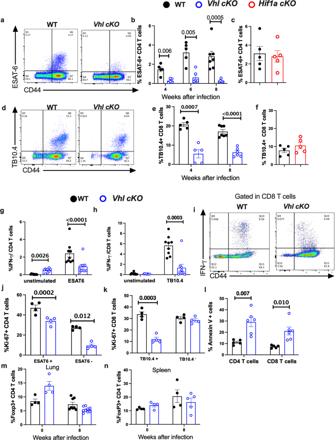Fig. 2: Reduced accumulation of mycobacteria-specific T cells in the lungs ofM. tuberculosisinfectedVhl cKOmice. aRepresentative dot plots of tetramer ESAT-6-binding CD4 T cells in the lungs fromVhl cKOand WT mice 8 weeks post infection (w.p.i.) withM. tuberculosisare depicted.bThe percentage of tetramer ESAT-6-binding CD4 T cells in the lungs ofVhl cKOand WT mice (WTn= 5, 5, 7 andVhl cKOn= 5, 7, 7 mice at 4, 6 and 8 w.p.i.) are displayed.cPercentage of tetramer ESAT-6 + CD4 T cells in the lungs ofHif1a cKO(n= 5) and WT (n= 5) mice 8 w.p.i. (d,e) Dot plots (d) and the frequency of tetramer TB10.4-binding CD8 T cells (e) in the lungs fromVhl cKO(n= 5, 6) and WT mice (n= 5, 7 animals at 4 and 8 w.p.i., respectively) are depicted.fThe frequency of tetramer TB10.4-binding lungHif1a cKO(n= 5) and WT (n= 5 mice) CD8 T cells at 8 w.p.i. is depicted.g,hThe frequencies of IFN-γ secreting CD4 (g) and CD8 (h) T cells fromVhl cKO(n= 9) and WT (n= 9) mice at 8 wp.i. stimulated with either ESAT-61-15or TB10.44-11peptides or left untreated are shown.iDot plots showing the IFN-γ secretion by lung CD8 T cells fromVhl cKOand WT mice 8 weeks afterM. tuberculosisinfection.j,kThe frequency of Ki-67 + , tetramer-binding and total CD4 (j) and CD8 (k) T cells from lung ofVhl cKO(n= 5) and WT mice (n= 5) 8 w.p.i.lThe fraction of lung Annexin V + CD4 and CD8 T cells fromVhl cKO(n= 5) and WT (n= 6) mice at 8 weeks afterM. tuberculosisinfection is shown.m,nThe percentage of Foxp3 + CD4 T cells in the lungs (m) and spleens (n) ofVhl cKOand WT mice at 0 and 8 w.p.i. (Vhl cKOn= 5, WTn= 4) is depicted (lungs 0 w.p.i. WTn= 4,Vhl cKOn= 4; 8 w.p.i. WTn= 5Vhl cKOn= 8; spleens 0 w.p.i.n= 4,Vhl cKOn= 4; 8 w.p.i WTn= 4,Vhl cKOn= 5). Each symbol represents one mouse, and the data are presented as the mean ± s.e.m. Thepvalues were calculated using a two-tailed unpairedttest with Welch’s correction and FDR adjustment for multiple comparisons. Source data are provided as a Source Data file. Then CD16/CD32 blocking antibodies (BD) and the fluorophore conjugated antibody cocktails (Supplementary Table 2 ) were introduced and incubated for 30 min on ice. Cells were then washed with PBS, resuspended and fixed with 2% paraformaldehyde solution in PBS. Data were acquired on a LSRII or a FACS Canto II flow cytometers controlled by a FACSDiva software version 6.0 and analyzed with FlowJo v10.7 (Tree star Inc., Ashland, OR). Examples of the gating strategies used are shown (Supplementary Fig. 10 ). Intravascular staining In some experiments, tissue-localized and blood-borne cells were discriminated by intravascular staining [73] . In short, mice were inoculated i.v. with 3 μg of FITC-labeled anti-CD45.2 (clone 104 BD), sacrificed 3–5 min after i.v. inoculation and lung cell suspensions were obtained and obtained as described above. Peripheral blood was sampled for every mouse as a positive control for i.v. labeling. Tetramer staining MHCII tetramers containing amino acids 1–20 of M. tuberculosis ESAT-6 or 240–254 of Ag85B and the MHCI tetramer containing amino acids 4–11 TB10.4 (all from the NIH Tetramer Core Facility, Atlanta, GA) were used for detection of M. tuberculosis -specific murine CD4 or CD8 T cells. Single-cell lung or MLN suspensions were stained at saturating concentrations with the tetramers and incubated at 37 °C for 1 h for the MHCII tetramers and at 4 o C for 30 min for the MHCI tetramer. Cells were then washed and stained with the fluorochrome antibody cocktails as described above. Intracellular staining For determination of IFN-γ-producing cells, spleen CD4 T cells were stimulated with either PMA/Ionomycin or anti-CD3/CD28, and lung cell suspensions from M. tuberculosis -infected mice were incubated with either 5 μg/ml ESAT6 1-15, 5 μg/ml TB10.4 4-11 or PMA/Ionomycin for 6 h at 37 o C. Brefeldin (10 μg/ml) was added to the cultures the last 4 h of stimulation. The IFN-γ secretion in naïve cells were then stained with live/dead staining followed by cell population-specific antibody cocktails. After labeling, cells were subsequently fixed and permeabilized using the leukocyte permeabilization reagent kit IntraPrep™ (Beckman, Brea, CA) and further stained with anti-IFN-γ (eBioscience, San Diego, CA). Data were acquired as described above. To determine the expression of CTLA-4, Foxp3 and Ki-67, cell suspensions were prepared as described above were fixed and permeabilized using the eBioscience FOXP3/Transcription Factor Staining Buffer Set (Invitrogen) according to the manufacturer’s protocol and stained with specific antibodies for FOXP3, Ki-67 and CTLA-4. To evaluate the expression of phospho-ribosomal protein S6, CD4 T cell suspensions were stained for surface markers as above, fixed with 2% PFA for 30 min on ice followed by permeabilization with Perm Buffer III (BD) for 30 min on ice. CFSE proliferation assay Cell suspensions were labeled in vitro with carboxyfluorescein succinimidyl ester (CFSE), to monitor distinct generations of proliferating cells by dye dilution. Prior to seeding, cells were labeled with 5 μM CFSE in PBS for 7 min and the reaction was stopped with 2 ml of ice cold 1% fetal calf serum (FCS) to absorb any unbound dye. Cell cycle profile and apoptosis assay To determine the cell cycle profile DNA was stained with propidium iodide. CD4 T cells were harvested, briefly vortexed to create a single cell suspension and fixed with 70% ethanol for 2 h on ice. Fixed cells were resuspended in PBS, washed twice, and treated with 100 µg/ml RNase A (Sigma) and 50 µg/ml propidium iodide before acquisition on the flow cytometer. Apoptosis was determined by Annexin V binding using FITC Annexin-V Apoptosis Detection Kit I (BD) according to supplier’s protocol. Cell suspensions were stained with surface markers and then incubated with 5 µL of PI and the Annexin V kit for 15 min at room temperature before analysis on the flow cytometer. Western blot CD4 T cells were sorted from lung cell suspensions from M. tuberculosis- infected mice by positive selection using MACS CD4 (L3T4) microbeads (Miltenyi Biotech). CD4 T cells either from infected mice or after stimulation in vitro with anti-CD3/CD28 were lysed in in RIPA buffer supplemented with protease and phosphatase inhibitor cocktail. Protein concentration was measured using BCA protein assay kit (Biorad) and 15 μg protein were and separated on 10% separating/5% stacking SDS-polyacrylamide gels. Samples were then transferred onto nitrocellulose membranes (BioRad, Hercules, CA) by electroblotting at 100 V, 250 mA for 80 min. 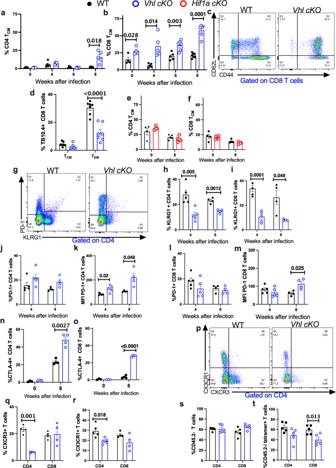Fig. 3: Decreased expression of differentiation markers and enhanced levels of inhibitory receptors inVhl cKOT cells duringM. tuberculosisinfection. a–cThe frequency of lung CD4 (a) and CD8 (b) TCM(CD44 + CD62L + ) fromVhl cKO(n= 4, 5, 6, 7) and WT (Vhl cKO; WTn= 4, 5, 5 and 7 mice at 0, 4, 6, and 8 weeks afterM. tuberculosisinfection are shown.cDot plot of CD44 and CD62L in lung CD8 T cells fromVhl cKOand WT mice 8 weeks after infection.dThe frequencies of tetramer TB10.4-binding pulmonary CD8 TCMand TEMcells fromVhl cKO(n= 6) and WT (n= 7) mice 8 weeks afterM. tuberculosisinfection are depicted.e,fThe fraction of pulmonary CD4 (e) and CD8 (f) TCMfromHif1a cKOand WT mice at 0 (n= 4 per group) and 8 (n= 5 per group) weeks afterM. tuberculosisinfection are depicted.g–mDot plots (g) and frequency of KLRG1 + and PD-1 + CD44 + CD4 (h,j) and CD8 (i,l) T cells in the lungs ofVhl cKOand WT mice at 4 and 8 weeks afterM. tuberculosisinfection. The MFI of PD-1 in CD4 (k) and CD8 T (m) cells in the lungs ofVhl cKOand WT mice is also shown (h–m;n= 5 and 4 mice per group at 4 and 8 weeks after infection).n,oThe fractions of CTLA-4 + CD4 (n) and CD8 (o) T cells in the lungs of mice before (n= 3) and 8 weeks (n= 4 mice per group) after infection are depicted.p–rDot plots (p) and frequencies of CXCR3+ (q) and CX3CR1+ (r) CD4 and CD8 T cells in the lungs ofVhl cKOand WT mice (n= 4 per group) 7 weeks afterM. tuberculosisinfection.s,tThe frequency of lung parenchymal (i.v. CD45.2 negative) total (s) and tetramer binding (t) CD4 and CD8 T cells in the lungs of WT andVhl cKOmice (n= 5 per group) 8 weeks after infection withM. tuberculosisare shown. Each symbol represents one mouse, and the data are presented as the mean ± s.e.m. Thepvalues were calculated using a two-tailed unpairedttest with Welch’s correction and FDR approach for multiple comparison. Source data are provided as a Source Data file. Immunostaining was performed using polyclonal rabbit anti-MYC or anti-HIF-1α or anti-actin (see Supplementary Table 3 for antibodies used). Membranes were then washed and incubated with horse-radish peroxidase-conjugated polyclonal goat anti-rabbit immunoglobulin and developed using ECL-Plus (Amersham Biosciences, Buckinghamshire, UK) and photographed using a Fuji intelligent dark box II digital camera. Histopathology The left lungs of mice infected with M. tuberculosis were dissected, fixed in 4% paraformaldehyde and embedded in paraffin. From each lung sample 4 15 μm sections were obtained and stained with hematoxylinn-eosin before evaluation. Real time-PCR Selected transcripts were quantified in lysates from CD4 T cells before or after in vitro anti CD3/CD28-stimulation by real time PCR as previously described [74] . Hprt was used as a control gene to calculate the ΔC t values for independent triplicate samples. The primer sequences used are displayed in Table S2 . The relative amounts of target/ hprt transcripts were calculated using the 2 −(ΔΔCt) method. These values were then used to calculate the fold increase of specific mRNA in CD4 T cells. RNA sequencing RNA was extracted from CD4 T cells obtained by positive selection from lungs of M. tuberculosis infected mice using CD4 Macs beads (Milteny) or from cultures of splenic CD4 T cells 24 h after stimulation with anti-CD3/CD28. RNA was isolated using miRNeasy micro kit (QIAGEN, Hilden, Germany) according to the manufacturer’s instructions and processed for sequencing at bioinformatics and expression analysis core facility (BEA) at Karolinska Institutet and at Novogene Biotech Co (UK). The RNA quality was assessed by 2200 TapeStation Instrument (Agilent, Santa Clara, CA). PolyA RNA selection was performed using the Illumina TruSeq RNA Sample Preparation Kit according to the manufacturer’s protocol. RNA-seq libraries were prepared and sequenced on the Illumina HiSeq 2000 platform at Bioinformatics and Expression Analysis core facility (BEA, Karolinska Institutet, Sweden). Preprocessed reads were aligned to the standard mouse reference genome mm10 using the HISAT2 program, and Hypergeometric Optimization of Motif EnRichment (HOMER, http://homer.salk.edu/homer ) was used to create the tag directory and count tags in all exons. For the gene expression analysis, unsupervised hierarchical clustering and principal component analysis of genes were performed in Qlucore Omics Explorer 3.2 (Qlucore, Lund, Sweden). Differentially expressed genes were determined by comparing groups using heteroscedastic two-tailed t tests. Multiple testing correction was performed using the Benjamini-Hochberg algorithm with a false discovery rate (FDR) of 1%. Gene Ontology enrichment analysis (Biological Process, Molecular Functions) or KEEG pathway enrichment was performed with WebGestalt ( http://www.webgestalt.org ) using default parameters. The raw and processed RNA sequencing data can be accessed at the GEO accession numbers GSE190791 and GSE190909. Statistics Statistical analysis and graphical representation of data were done using GraphPad Prism 9 software version 3(GraphPad Prism, San Diego, CA). We have used the unpaired t -test with Welch’s correction which assumes normal distribution but can be used when the two samples have unequal variances, and used a False discovery rate approach for multiple comparisons. 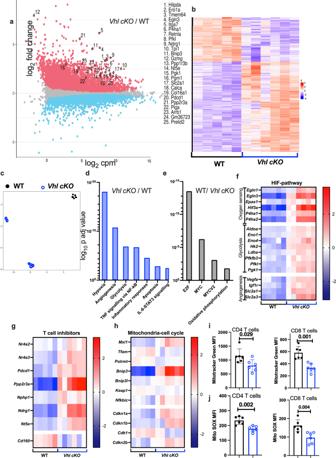Fig. 4: VHL expression in lung CD4 T cells fromM. tuberculosis-infected mice controls proliferation and effector responses. RNA seq was performed inVhl cKO(n= 6) and WT (n= 5) CD4 T cells isolated from the lungs ofM. tuberculosis-infected mice.aMA plot in which each point represents a gene. The plot illustrates the change of expression (yaxis, log2fold change) and the average transcript abundance over all samples (xaxis, log2counts per million). Colors indicate the significantly upregulated (in red) or down-regulated (in light blue) inVhl cKOas compared to WT CD4 T cells. The top 25 most significant genes are indicated by their gene symbols.bIn the heat map the log2counts for each gene (row) is standardized to mean = 0, and the differences with the mean depicted.cUmap dimensionality reduction plots from non-supervised samples based on the normalized gene counts after filtering the low expressed genes. There are 2 outliers in theVhl cKOCD4 T cell group, probably explained by their lower sample weight.d,eThe log10pvalue of the enrichment of hallmark gene sets in the transcriptome ofVhl cKO(d) and WT (e) CD4 T cells was compared using the MSigDB databases.f–hThe heat maps of selected RNA-seq data showing: HIF-pathway-specific genes (f), genes involved in T cell exhaustion or dysfunction (g), and MYC-regulated transcripts (h). Data were normalized by subtracting the log2transformed values to the mean log2value for all samples for each gene.i,jLung cell suspensions were labeled with mitochondrial-selective MitoTracker Green to assess mitochondrial mass and Mito Tracker Red to measure mitochondrial ROS. The MFI of Mito Tracker green, to assess mitochondrial mass (i), and Mito SOX Red, to assess mitochondrial ROS, (j) labeled live CD4 and CD8 T cells from the lung ofVhl cKOand WT mice (n= 6 per group) 8 weeks after infection withM. tuberculosisare shown.i,jEach symbol represents one mouse, and the data are presented as the mean ± s.e.m.d–jThepvalues were calculated using a two-tailed unpairedttest with Welch’s correction (k,m) and FDR adjustment for multiple comparisons (d–h). Source data are provided as a Source Data file. 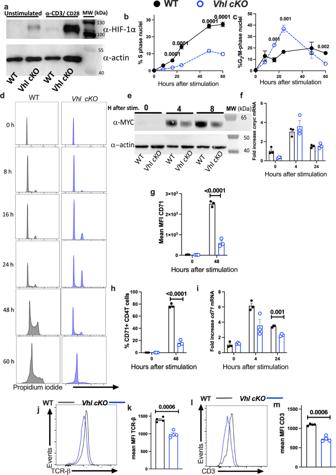Fig. 5: VHL expression is required for TCR activation of CD4 T cells. aNaïve CD4 T cells were enriched by negative selection fromVhl cKOand WT spleens and stimulated with anti-CD3/CD28. Cell lysates were analysed by Western blot before and after TCR stimulation using anti-HIF-1α and anti-β-actin antibodies. One of three independent similar experiments is shown.b–dThe mean % of S-phase (b) and G2/M (c) CD4 T cells and representative histograms (d) of the cellular DNA content after propidium iodide staining ofVhl cKOand WT CD4 T cells at different times after anti-CD3/CD28 stimulation are shown.eCell lysates fromVhl cKOand WT CD4 T cells were analysed by immunoblot after anti-CD3/CD28 stimulation using anti-MYC or anti-β-actin antibodies. One representative of two independent experiments is shown.fTotal RNA was extracted fromVhl cKOand WT CD4T cells at different times points after anti-CD3/CD28 stimulation.CmycmRNA titer was normalized toHprtmRNA levels in the same samples. TheCmycmRNA fold increase levels are depicted.g,hThe frequency (h) and expression level (g) of CD71 inVhl cKOand WT CD4T cells are shown.iThe fold change levels ofcd71mRNA inVhl cKOand WT CD4 T cells was determined by real time-PCR.j–mRepresentative histograms and the MFI of the TCR-β (j,k) and CD3 (l,m) expression inVhl cKOand WT CD4 T cells are shown. Each symbol represents one independent sample, and the data are presented as the mean ± SEM. n = 3 (b,c,f–i), andn= 4 (k,m).p-values were calculated using a two-way ANOVA (b,c) or a two-tailed unpairedttest with Welch’s correction and a FDR adjustment (f–i,k,m). Source data are provided as a Source Data file. We have two way ANOVA with a Sidak correction for multiple comparisons of the same parameters (for example for analyzing kinetics). Bacterial titers were log 10 -transformed for normalization. Statistical significance between three or more groups was determined using one- or two-way ANOVA. The in vitro experiments are performed with triplicate biological replicates and each experiment was repeated at least twice. The bar plots showing the mean and error bars have symbols that denote the individual values. 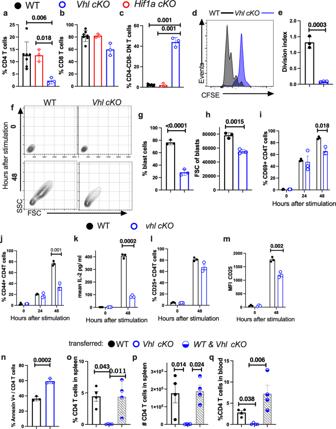Fig. 6: VHL promotes proliferation of CD4 T cells in response to TCR activation. a–cThe % CD4 (a), CD8 (b) and DN (c) T cells inVhl cKO(n= 3),Hif1a cKO(n= 3) and WT (n= 6) spleen cell suspensions measured 6 days after anti-CD3/CD28 stimulation is shown.dRepresentative histogram of CFSE-labeledVhl cKOand WT CD4 T cells 3 days after stimulation with anti-CD3/CD28 are shown.eThe CFSE labeling was used to calculate the division index (the average number of cell division that a cell in the original population has undergone).f–hDot plots showing the FCS/SSC of lymphocyte gatedVhl cKOand WT CD4 T cells before and 48 h after stimulation with anti-CD3/CD28 (f). The mean percentage of blast cells (g) and the FSC of blasts (h) 48 h after anti-CD3/CD8 stimulation are shown.i,jThe percentage of CD69+ (i) and CD44 +  (j)Vhl cKOand WT CD4 T cells after anti-CD3/CD28 stimulation are depicted.kThe titers of IL-2 in the culture supernatants fromVhl cKOand WT CD4 T cells before and 48 h after anti-CD3/CD28 stimulation.l,mThe percentage of cells expressing CD25 (l) and the MFI of CD25 (m) on TCR-stimulatedVhl cKOand WT CD4 T cells is depicted.nThe percentage of Annexin V +Vhl cKOand WT CD44 + CD4 T cells 3 days after stimulation with anti-CD3/CD28.e,g–nn= 3 independent cultures per group.o,pRag2−/−mice were transferred i.v. with either 2.106CD4 T cells from CD45.2Vhl cKO, CD45.1 WT or a mixed 1:1 suspension from both genotypes (106cells/each). The percentages and numbers of CD4 T cells in the spleen (o,p) and blood (q) of mice 5 weeks after transfer is shown (n= 4 mice per group). Each symbol represents one independent biological sample, and the data are presented as the mean ± SEM.p-values were analysed using two-tail unpairedttest (e,g–n) with FDR adjustment or one-way ANOVA with Welch’s correction (a–c,o–q). Source data are provided as a Source Data file. 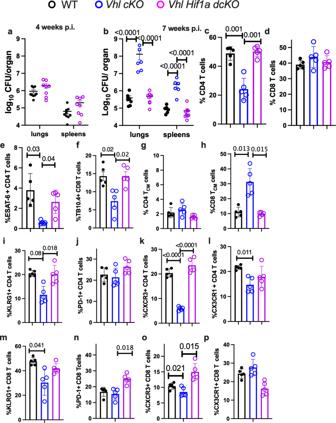Fig. 7: HIF-1 mediates the susceptibility toM. tuberculosis-infection ofVhl cKOmice. a,bVhl cKO, Vhl Hif1a dcKOand WT mice were sacrificed at 4 (a) and 7 (b) weeks after aerosol infection withM. tuberculosis. The log10CFU in lungs and spleens are depicted; (a) WTn= 9,Vhl Hif1a dcKOn= 8, (b) WTn= 6,Vhl cKOn= 6,Vhl Hif1a dcKOn= 9.c,dThe frequency of CD4 (c) and CD8 (d) T cells in the lung ofVhl Hif1a dcKO,Vhl cKOand WT mice 7 weeks afterM. tuberculosisinfection is shown.e,fThe percentage of tetramer ESAT-6-binding CD4 T cells (e) and TB10.4-binding CD8 T cells (f) in the lung ofVhl Hif1a dcKO,Vhl cKOand WT mice 7 weeks after infection are displayed.g,hThe frequency of CD4 (g) and CD8 (h) TCMin the lung ofVhl cKO, Vhl Hif1a dcKOand WT mice 7 weeks afterM. tuberculosisinfection is shown.i–pThe frequency of KLRG1 +  (i,m), PD-1 +  (j,n), CXCR3 +  (k,o) and CX3CR1 +  (l,p) CD4 and CD8 T cells in the lung ofVhl Hif1a dcKO,Vhl cKOand WT mice 7 weeks after infection withM. tuberculosis.c–pn= 5 mice per group. Each symbol represents one mouse, and the data are presented as the mean ± SEM.p-values were calculated using one-way ANOVA test with Welch’s correction for unequal SD and Dunnet’s T3 adjustment for multiple comparisons. Source data are provided as a Source Data file. 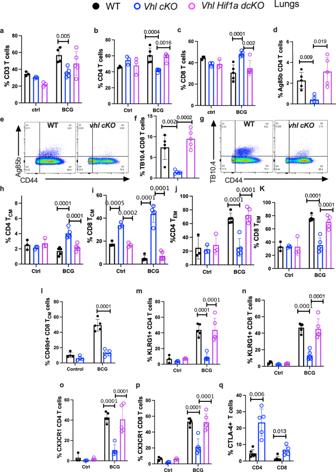Fig. 8: HIF-1 stabilization in T cells impairs the responses to immunization with BCG. a–cThe frequency of total (a), CD4 (b) and CD8 (c) T cell populations in lungs before and 3 weeks after i.v. immunization with BCG are depicted.d–gThe percentages (d,f) and representative dot plots (e,g) of tetramer Ag85b-binding CD4 T cells (d,e) and TB10.4 tetramer-binding CD8 T cells (f,g) in the lungs ofVhl Hif1a dcKO,Vhl cKOand WT mice (n= 5 per group) after BCG immunization are shown. The frequencies of TCM(h,i), TEM(j,k) in CD4 and CD8 T cells in lungs fromVhl Hif1a dcKO,Vhl cKOand WT mice at 0 or 3 weeks after BCG immunization are depicted.lThe percentage of lung CD49d + CD8 TCMbefore and after BCG immunization of WT andVhl cKOmice are shown. The frequencies of KLRG1 +  (m,n) and CX3CR1 +  (o,p) in CD4 and CD8 T cells in lungs fromVhl Hif1a dcKO,Vhl cKOand WT mice at 0 or 3 weeks after BCG immunization are depicted.qThe fraction of CTLA-4 + CD4 and CD8 T cells in the lung of BCG immunized mice are shown. Each symbol represents one mouse, and the data are presented as the mean ± SEM (a–k,m–p) before immunizationn= 3 per mice per group, after immunizationn= 5 per group;lbeforen= 4 per group, after immunizationn= 5 per group;qn= 5 per group.p-values were calculated using 2-way ANOVA test, with Sidak adjustment for multiple comparisons. Source data are provided as a Source Data file. 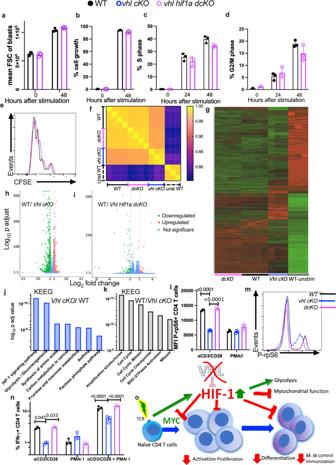Fig. 9: HIF-1 stabilization impairs CD4 T cell responses in vitro. a,bThe FSC of blasts (a) and the % cell size increase relative to unstimulated cells in the blast population (b) were depicted.c,dThe % of S-phase (c) and G2/M (d) of CD4 T cells are shown.eCFSE profiles ofVhl Hif1a dcKOand WT CD4 T cells 3 days after stimulation with anti-CD3/CD28 are shown.f–mRNA-seq was performed in independent cultures of WT (n= 4),Vhl cKO(n= 3) andVhl Hif1a dcKOCD4 T (n= 4) cells before or 24 h after anti CD3/CD28 stimulation.fThe Pearsson R2correlation matrix of the expression of all genes in each sample is shown.gHeat map of the log2counts for each gene standardized to the mean.h,iVolcano plots showing the log2fold change in gene expression (x-axis) andp-value (y-axis), of differentially upregulated or downregulated genes (p≤ 0.05 and log2fold change > 1) (i).j,kThe log10pvalue of the most enriched KEEG-pathway terms inVhl cKOvs WT (j) or in WT vsVhl cKOCD4 T cells (k).l,mThe MFI (l) and a representative histogram (m) of phospho-rpS6 onWTand mutant CD4 T cells 2 h after anti-CD3/CD28 or PMA/I stimulation are illustrated.nThe frequency of IFN-γ expressing WT,Vhl cKOandVhl Hif1a dcKOCD4 T cells 6 h after PMA/I or 72 h after anti-CD3/CD28 stimulation are shown. A group was stimulated with anti-CD3/CD28 for 65 h and then incubated for 6 h with PMA/I.a–d,l,nEach symbol represents one independent sample (n= 3 per group), and the data are presented as the mean ± SEM.p-values were calculated using a two-tailed unpairedttest with Welch’s correction (a–d) and 2-way ANOVA test, with Sidak adjustment for multiple comparisons (l,n). Source data are provided as a Source Data file.oVHL promotes the cell cycle progression, growth responses, proliferation, IL-2 secretion and expression of activation markers of TCR-stimulated CD4 T cells, the differentiation and the protective function of T cells againstM. tuberculosisinfection as well as the responses to immunization by impairing HIF-1 stabilization. Reporting summary Further information on research design is available in the Nature Research Reporting Summary linked to this article.